Fano resonances and all-optical switching in a resonantly coupled plasmonic–atomic system The possibility of combining atomic and plasmonic resonances opens new avenues for tailoring the spectral properties of materials. Following the rapid progress in the field of plasmonics, it is now possible to confine light to unprecedented nanometre dimensions, enhancing light–matter interactions at the nanoscale. However, the resonant coupling between the relatively broad plasmonic resonance and the ultra-narrow fundamental atomic line remains challenging. Here we demonstrate a resonantly coupled plasmonic–atomic platform consisting of a surface plasmon resonance and rubidium ( 85 Rb) atomic vapour. Taking advantage of the Fano interplay between the atomic and plasmonic resonances, we are able to control the lineshape and the dispersion of this hybrid system. Furthermore, by exploiting the plasmonic enhancement of light–matter interactions, we demonstrate all-optical control of the Fano resonance by introducing an additional pump beam. Resonantly coupled photonic systems exhibiting dispersive and nontrivial line shapes are attracting growing attention in recent years. In particular, light–matter interactions are of interest owing to both their basic physical properties as well as their potential applications. Furthermore, with the emergence of plasmonics structures and devices that are capable of confining light to the deep sub wavelength regime, it is now possible to enhance light–matter interactions at the nanoscale. Therefore, fascinating phenomena such as atomic transition lifetime shortening and enhanced spontaneous emission [1] , stronger nonlinear interactions [2] and slow light effects [3] can now be readily observed. Systems supporting such coupling are of major importance in science and technology, as their properties can vary drastically depending on the coupling conditions. Two universal effects that may arise by the resonant coupling of atoms and plasmons are the Fano spectral lineshape [4] , [5] , [6] , [7] , [8] , [9] , [10] , [11] , [12] , [13] , [14] and the resonance splitting [15] , [16] , [17] , [18] , [19] , the latter being attributed to strong coupling. While the original work of Fano [4] describes the coupling between an atomic resonance and the continuum, nowadays it is common to use a broader definition in which a narrow resonant line width system is coupled to a system with a broader resonance. A major interest in studying such coupled resonant systems is the ability to precisely control its lineshape. For example, the same system can provide symmetric, antisymmetric and asymmetric lineshape, depending not only on the inherent properties of each resonance, but primarily on their relative frequency separation. Over the years, Fano resonances have been studied theoretically and experimentally in a variety of photonic systems [5] , [6] , [7] . Due to the high sensitivity to variations in refractive index, devices exploiting Fano resonances are excellent candidates to mitigate applications such as sensing and switching [7] , [8] . More recently, Fano resonances were also observed in several plasmonic systems initiating a flourishing research in the field [9] , [10] , [11] , [12] , [13] , [14] . In particular, Fano resonances in coupled plasmonic–molecular systems have been observed in systems of localized plasmons interacting with molecular vibrational modes [13] , [14] . It would therefore be of great interest to further explore such effects in a hybrid plasmonic–atomic system, where a collection of single atoms is resonantly hybridized with the highly confined plasmons. The use of a metal layer adjacent to alkali vapours has been exploited for the study of optical forces that the evanescent plasmonic field exerts on alkali vapours [20] , [21] . Furthermore, Chevrollier et al. [22] have used a thin gold layer to observe reflection atomic spectroscopy of light impinging on the metal–vapour interface at normal incidence. Investigating the coupled resonant interaction between surface plasmonic polaritons and atomic vapour is interesting from a fundamental light–matter interaction perspective, and it may also serve to inform other studies of plasmonic–atomic resonant interactions. In particular,, by exploiting the unprecedented field enhancement in plasmonic structures, nonlinear interactions may be enhanced to remarkable levels [23] . In this context, one should mention that enhancing the interaction of light with thermal alkali vapours can also be achieved by using photonic-guided modes, as demonstrated in hollow core photonic crystal fibres [24] , [25] , hollow core anti-reflecting optical waveguides [26] , [27] , and tapered nanofibres [28] , [29] . Recently we have realized the platform of an atomic cladding waveguide consisting of chip-scale nano waveguides integrated with rubidium (Rb) cladding. Using this approach, we have demonstrated light–matter interactions on a chip, with nanoscale dimensions and low light level linear and nonlinear interactions [30] . These efforts towards miniaturization and integration of light–vapour systems may be further motivated by using integrated plasmonic structures with the benefit of extreme light confinement. Having metals in the vicinity of the vapours could play a positive role in adding new functionalities such as localized heating, and applying electrostatic or magnetic fields. Motivated by this interest in resonant coupling between plasmonic and atomic systems, we study the interactions between a surface plasmon resonance and Rb vapour. We show that due to the Fano interplay between the atomic and the plasmonic resonance, having five orders of magnitude difference in their spectral line widths, the resonance of the combined system may vary drastically by changing the coupling conditions. The experimental results are explained by a model which takes into account the plasmonic resonance, as well as the finite light–matter interaction time resulting from the strong-mode confinement and the motion of the atoms. As an example for a potential application, we demonstrate the capability for all-optical control of the Fano resonance. Taking advantage of the plasmonic enhancement of light–matter interactions, we were able to switch off the Fano fingerprint and obtain a nearly flat spectral response. Construction of the hybrid plasmonic–atomic device Our hybrid plasmonic–atomic device is illustrated schematically in Fig. 1a . The light beam is coupled to a surface plasmon polariton (SPP) mode propagating at the interface between the metal and the atoms. As a consequence, the atoms interact with the evanescent tail of the SPP mode. The device consists of a glass prism coated by a 3-nm adhesion layer of Ti, and a 42-nm layer of Au. Finally, a 5-nm layer of MgF 2 is evaporated on top of the Au layer for the purpose of protecting the metal from interacting with the Rb atoms. A glass (Pyrex) cylinder is then bonded to the chip using thermal-cured epoxy glue. Next, the atomic cell is baked out to a vacuum level better than 10 −7 Torr, and a droplet of 85 Rb is inserted. Finally the cylinder is pinched off. As a result, a portable and stand-alone device is constructed. A photograph of a bare plasmonic prism and the hybrid plasmonic–atomic device is presented in Fig. 1b . We excite the SPP mode using the well-known Kretschmann configuration (a schematic representation of the experimental setup is given in Fig. 1c ). To interrogate the D2 line of Rb, we use a 780-nm laser with an ~1 mm collimated beam. The atomic cell is heated by resistive heaters to approximately 60 °C, defining the cold spot of the device. We keep the cold spot away from the metal to protect it from condensation of Rb. The power level of the signal was kept in the range of 1 μW. 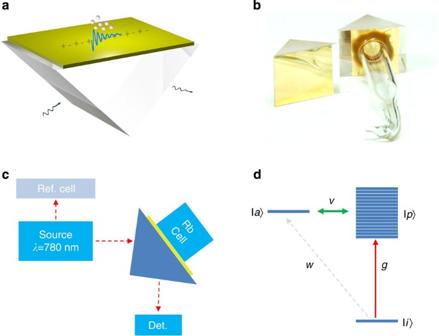Figure 1: Plasmonic–atomic integrated-coupled system. (a) Illustration of the plasmonic–atomic device consisting of a glass prism, covered by a stack of 3-nm-thick Ti layer, 42-nm-thick gold layer and 5-nm-thick MgF2layer bonded to an atomic vapour cell. (b) Photograph of the bare plasmonic prism and the plasmonic–atomic device. (c) Schematic representation of the experimental setup. (d) Level scheme schematics of plasmonic–atomic-coupled system. Here, level |i> represents the incident state, coupled directly to the plasmonic broad state |p> with a coupling strengthg. The coupling between the plasmonic state and the discrete atomic state |a> is also possible with a coupling coefficientv. Finally, an indirect coupling may be achieved through the incident level to the atom with a coupling coefficientw. Figure 1: Plasmonic–atomic integrated-coupled system. ( a ) Illustration of the plasmonic–atomic device consisting of a glass prism, covered by a stack of 3-nm-thick Ti layer, 42-nm-thick gold layer and 5-nm-thick MgF 2 layer bonded to an atomic vapour cell. ( b ) Photograph of the bare plasmonic prism and the plasmonic–atomic device. ( c ) Schematic representation of the experimental setup. ( d ) Level scheme schematics of plasmonic–atomic-coupled system. Here, level | i > represents the incident state, coupled directly to the plasmonic broad state | p > with a coupling strength g . The coupling between the plasmonic state and the discrete atomic state | a > is also possible with a coupling coefficient v . Finally, an indirect coupling may be achieved through the incident level to the atom with a coupling coefficient w . Full size image Modelling the transmission through the hybrid device As mentioned before, a hybridized-coupled system consisting of a broad resonance and a narrow resonance gives rise to a Fano lineshape. In the original work of Fano, the atomic levels were coupled to the continuum representing the discrete and the broad resonances, respectively. Applying the Fano formalism to our atomic–plasmonic system leads to the same qualitative behaviour, where the broad plasmonic resonance replaces the continuum modes [12] . We describe such a scheme in Fig. 1d , where | i ›, | p › and | a › are the incident state, plasmonic states and atomic state, respectively. Here, v represents the evanescently mediated coupling between the atomic state and the plasmonic continuum, w represents the direct coupling of light to the atomic state, and g represents the direct coupling to the plasmonic system. By solving the Hamiltonian governing this coupled system (ref. 12 ), one obtains the canonical form of Fano lineshape, namely: where q =2 vw /( g Γ d ( E ))+2Δ/Γ p and e =2 E /Γ d ( E )−2Δ/Γ p . Here, Γ d ( E ) is related to the spectral width of the discrete state, Γ p is the spectral width of the plasmonic resonance and Δ is the energy difference between the plasmonic resonance and the excitation energy E . In our experiment, this energy E is scanned in the proximity of the atomic resonance, and thus Δ is approximately the energy difference between the plasmonic and atomic resonance. The q parameter governs the symmetry of the lineshape, where four distinct regimes are identified: q=∞, corresponding to a Lorentzian line shape; q= 0, corresponding to an inverted symmetric Lorentzian line shape; q> 0 anomalous dispersion-like antisymmetric and asymmetric line shapes; q< 0, normal dispersion-like antisymmetric and asymmetric line shapes. Truly symmetric lines are achieved when q is equal to zero. By observing this scenario for the case of very small values of Δ, one may deduce that w →0 and thus the coupling of light into the atomic states occurs only via the indirect route (that is, via the plasmonic system). While the Fano model provides an excellent physical insight regarding the nature of the coupled system, we now turn into a semiclassical description to further quantify the transmission of light propagating through our hybrid system. With this approach, it is easier to take into account the exact lineshape of the plasmonic and the atomic system, as well as to account for the loss mechanisms. This approach was shown to be useful and adequate for many Fano systems, for example [6] , [31] , [32] , [33] . We start by adapting the formalism of attenuated total internal reflection [34] , [35] , [36] , [37] and modify it to account for our configuration. First, one needs to find the effective susceptibility of the atomic media, taking into account the motion of the atoms, their quenching on the surface and the wave vectors of the evanescent radiation. As such, it includes two broadening mechanisms: enhanced (relative to vacuum) Doppler broadening and transit time broadening. A detailed description of the procedure is given in ref. 30 . To calculate the effective susceptibility, we need to find the wave vectors describing the SPP mode. To do so, we use a three-layer model, representing the glass prism, the metal (with realistic value of relative permittivity of −24+i6) and the air. This procedure is perturbative in its nature, as it neglects the effect of the Rb atoms on wave vectors of the SPP mode. Yet, it can be easily justified because of the low density of the atoms, and it was already shown to provide excellent match to experimental results [30] , [34] , [35] , [36] , [37] . Based on this procedure, we find the evanescent decay length and the effective index of the SPP mode at the wavelength of 780 nm to be ~500 nm and 1.03, respectively. Using these wave vectors, we calculate the effective atomic susceptibility, with density of atoms corresponding to 60 °C. We plot the imaginary and the real part of the effective index (using the relation n =(1+ χ ) 1/2 ) as a function of the frequency detuning in Fig. 2a,b , respectively. The line width (full width half maximum) of a single atomic transition, according to this model is ~610 MHz. This line width is the result of two major broadening mechanisms: first, Doppler broadening, that is, Δ ω = k·v atoms , which is approximately 570 MHz (we have used the plasmonic k -vector, which is slightly larger than the free-space k-vector); and second, transit time broadening of approximately 40 MHz. One should note that the full width half maximum of the line observed in Fig. 2a appears to be slightly larger (~640 MHz). This is because of the upper hyperfine atomic transitions which cannot be easily resolved. 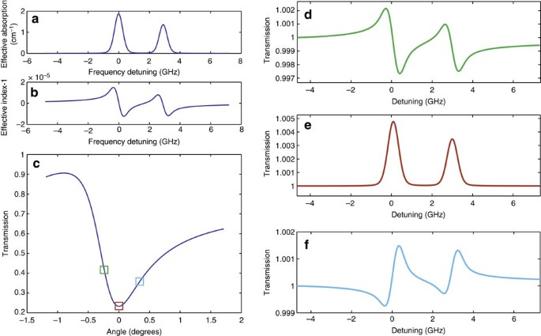Figure 2: Calculated transmission of plasmonic–atomic system. (a) Calculated effective imaginary index of refraction of rubidium. (b) Calculated effective real index of refraction of rubidium. (c) Calculated transmission of ‘bare’ plasmonic system around the resonance, as a function of the excitation angle (relative to plasmonic resonance angle) using a three-layer model. (d–f) Calculated transmission of the combined atomic–plasmonic system at an angle corresponding to the green, red and blue square marks inFig. 2c, respectively. Figure 2: Calculated transmission of plasmonic–atomic system. ( a ) Calculated effective imaginary index of refraction of rubidium. ( b ) Calculated effective real index of refraction of rubidium. ( c ) Calculated transmission of ‘bare’ plasmonic system around the resonance, as a function of the excitation angle (relative to plasmonic resonance angle) using a three-layer model. ( d – f ) Calculated transmission of the combined atomic–plasmonic system at an angle corresponding to the green, red and blue square marks in Fig. 2c , respectively. Full size image Next, we allocate the obtained value of effective susceptibility to the atomic layer, and use the three-layer model, to find the combined transmission of the plasmonic–atomic system. To better explain our results, we first plot ( Fig. 2c ) the ‘bare’ plasmonic resonance (neglecting the atomic effects) as a function of the incident excitation angle. We refer to three distinct regimes (as denoted by the square marks) in which the excitation angle is smaller (green), equal (red) or larger (blue) than the angle of resonance. We now plot the combined transmission of our hybrid plasmonic–atomic system, at each of these regimes, in Fig. 2d (green) Fig. 2e (red) and Fig. 2f (blue). A Fano lineshape is clearly observed. Typically to the Fano effect, one can observe the transition of the transmission curve from anomalous dispersion regime ( Fig. 2d ) through the nondispersive regime (symmetric lineshape, Fig. 2e ) towards the normal dispersive regime ( Fig. 2f ). In reference to the previous discussion regarding the q parameter in the original Fano model, these corresponded to q parameters of 0.6, 0 and −0.6, respectively. As a consequence, our system offers the flexibility of choosing the dispersive nature of the transmission function by controlling the momentum of the excitation source. This is achieved by controlling a ‘knob’, that is, the angle of excitation. The immediate application that may benefit from this feature is the use of the dispersive signal directly as an error signal for frequency locking. Measuring the transmission of the combined system Next, we describe the experimental results of our hybrid plasmonic–atomic system. First, we measure the transmission around the plasmonic resonance, neglecting the influence of the atoms. This can be achieved, for example, by selecting a wavelength which is slightly detuned from the atomic resonances and scan the transmission of the system as a function of incident angle ( Fig. 3a ). In Fig. 3b , we show the measured transmission spectrum of our plasmonic–atomic device (blue lines). As a reference, we have recorded simultaneously the absorption lines using a different Rb cell, containing natural Rb (and hence the additional dip of 87 Rb in the reference data). The measured reference and signal are presented on the same scale in Fig. 3b (green-dashed lines). Each panel shown in Fig. 3b is obtained at a different incident angle, corresponding to a different coupling condition to the plasmonic resonance, where the dip of the plasmonic resonance is obtained at ~43°, marked as 0°. 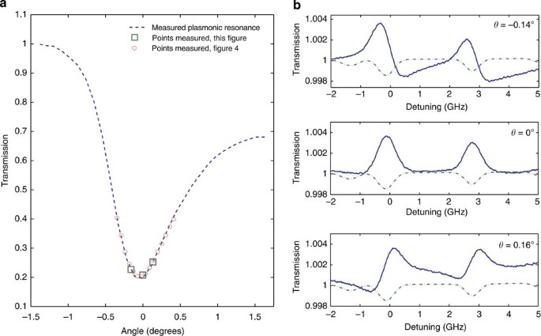Figure 3: Transmission spectra of the plasmonic–atomic device. (a) Measured plasmonic resonance. The blue-dashed line represents the measured plasmonic resonance over a broad angular range. We mark distinct angles by red and green squares. Each green square refer to a different panel inFig. 3b, whereas each red circle refers to a different panel presented later, inFig. 4. (b) Transmission as a function of frequency detuning for different angles of incidence (blue solid line). Transmission through a reference cell of natural Rb is presented by the dashed green lines. Figure 3: Transmission spectra of the plasmonic–atomic device. ( a ) Measured plasmonic resonance. The blue-dashed line represents the measured plasmonic resonance over a broad angular range. We mark distinct angles by red and green squares. Each green square refer to a different panel in Fig. 3b , whereas each red circle refers to a different panel presented later, in Fig. 4 . ( b ) Transmission as a function of frequency detuning for different angles of incidence (blue solid line). Transmission through a reference cell of natural Rb is presented by the dashed green lines. Full size image Clearly, one can see a striking resemblance between the predicted ( Fig. 2c–f ) and the measured transmission. Starting at an angle of −0.14 ° we obtain an anomalous dispersion curve, which is gradually evolves towards a symmetric transmission peak at an angle of 0 ° . By further increasing the angle towards 0.16 ° , a normal dispersion curve is observed. These observed results serve as a clear indication of a Fano effect. Once again, being able to control the plasmonic resonance using the ‘knob’ of incident angle, provide us with an excellent tool to study the nature of this combined system and to precisely control its transmission spectrum. To further investigate the evolution of Fano interference in our hybrid plasmonic–atomic structure, we now specifically focus on the F =3 to F ′=2/3/4 85 Rb transition. As before, we plot ( Fig. 4 ) the transmission as a function of the frequency detuning. This time, the results are measured over a wider range of angles spanning approximately 1 ° around the plasmonic resonance, and the angular resolution is set to ~0.05 ° to show the full evolution of the Fano effect. 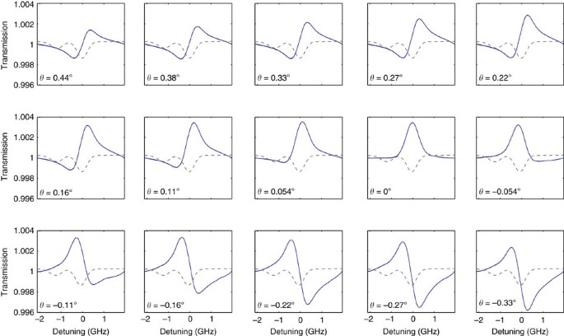Figure 4: Evolution of the Fano resonance in the plasmonic–atomic device Transmission as a function of frequency detuning for different angles of incidence (blue solid line), and reference absorption lines (green dashed). Figure 4: Evolution of the Fano resonance in the plasmonic–atomic device Transmission as a function of frequency detuning for different angles of incidence (blue solid line), and reference absorption lines (green dashed). Full size image Here, one can clearly observe the gradual transition between the antisymmetric anomalous dispersion line ( θ =0.44°), where the midslope coincides with the atomic reference resonance, through an asymmetric line (for example, θ =0.33 ° , θ =0.27 ° ), towards a symmetric peak obtained at θ =0°. A mirror behaviour is observed for angles left of the plasmonic resonance, however, the contrast of the measured signal is larger (for instance in θ =−0.27 ° ) as compared with the dispersion line obtained after the plasmonic resonance. This observation can be explained by the asymmetry of the plasmonic resonance. Apart from the above analysis as a Fano resonance, the obtained results can be analysed in the context of a plasmonic sensor of refractive index. With this approach, modifying the real and imaginary indices of refraction of the top layer induces a change in the transmission. However, for each incident angle, the transmission sensitivity, that is, the amount of change in transmission as a result of a small variation in the imaginary and the real part of the refractive index, is different. For instance, at an angle of −0.3° with respect to the plasmonic resonance, transmission changes (with respect to the bare plasmonic resonance) of about 0.1% or 0.02% are obtained for 10 −3 change in the real or the imaginary parts of the refractive index, respectively. In contrast, at an angle of 0°, the transmission varies by 0.5% or 5% for the same value of 10 −3 change in the real or the imaginary parts of the refractive index, respectively. From these results we identify two conclusions. First, the sensitivity in general is larger around resonance. Furthermore, while around resonance the transmission is mostly affected by a change in the imaginary part of the refractive index, this trend is inverted as we move away from resonance. The measured line width, at 0 ° for which both the atomic and plasmonic resonance coincide is 710 MHz, which is larger than the theoretical line width of 640 MHz mentioned earlier. The difference can be attributed to calibration inaccuracies and perhaps more interestingly to additional surface-broadening mechanisms arising from the metal–vapour interface, such as van der Waals interactions [38] , [39] . Such effects will be studied in detail in the future. We now compare the measured results presented in Fig. 4 to the theoretical model. To do so, we first fit the theoretical plasmonic resonance, to the measured one by using a five-layer model, including the Ti adhesion layer, and the MgF 2 -protecting layer. We do so by varying a single parameter—the thickness of the gold layer (within 5% of the designed thickness value). Next, we use the effective susceptibility of the Rb atoms (using the simulated parameters of the SPP, and the measured temperature of ~60 ° C) and incorporate it as the top medium in the five-layer model. We plot the measured and the theoretical transmissions in Fig. 5a,b , respectively. 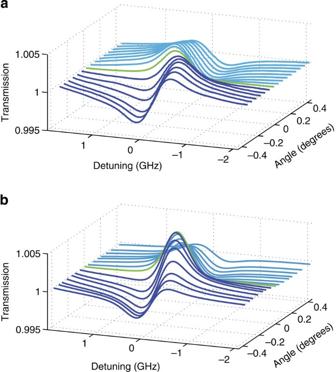Figure 5: Hybrid device transmission spectra compared with theory. (a) Measured and (b) calculated transmission as function of frequency detuning for different angles of incidence. Figure 5: Hybrid device transmission spectra compared with theory. ( a ) Measured and ( b ) calculated transmission as function of frequency detuning for different angles of incidence. Full size image As can be seen, the model predicts the transmission of the hybrid plasmonic–atomic system both qualitatively and quantitatively. Both the contrast and, as mentioned earlier, the width of the atomic resonance are predicted quite accurately, as well as the dispersive characteristics around the plasmonic resonance. However, the transition from anomalous dispersion through symmetric lineshape to normal dispersion occurs faster in the measurement as compare with our simulations. This may be due to a difference between the modelled and the measured plasmonic resonance lineshape. All-optical control over Fano line shapes Finally, we investigate and demonstrate the ability to control the Fano resonance using another optical beam. By doing so, it is possible to manipulate the lineshape and the extinction of the Fano resonance. As a consequence, one can optically manipulate both the absorption and the time delay properties of the probe beam. Our experimental arrangement is presented in Fig. 6a . We excite the plasmonic–atomic system by using two different wavelengths: a pump at the wavelength 780 nm, and a probe at the wavelength of 795 nm. Once combined using beam splitter, the two beams copropagate and pass simultaneously through a reference cell, and the plasmonic–atomic hybrid device. Finally, the pump beam is filtered out using a grating and is detected using a photodiode. 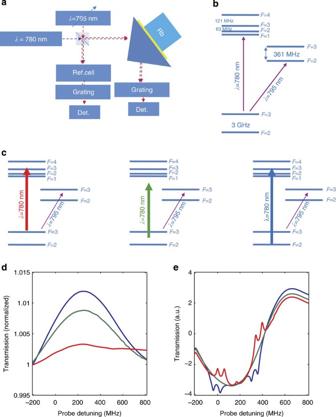Figure 6: All-optical switching of Fano line shapes. (a) Experimental setup. (b)85Rb-relevant transitions of the D1 and D2 manifolds (not to scale). (c) Illustration of three different pump scenarios. (d) Probe transmission as function of probe detuning for the three different pump scenarios described inc, through the plasmonic–atomic device. (e) Probe transmission through the reference cell. In both panels (d,e), the green line represents the case where the pump beam is tuned far from resonance, the blue line represents the pump beam tuned to theF=2 toF′ manifold, and the red lines represent tuning the pump toF=3 toF′ manifold. Figure 6: All-optical switching of Fano line shapes. ( a ) Experimental setup. ( b ) 85 Rb-relevant transitions of the D1 and D2 manifolds (not to scale). ( c ) Illustration of three different pump scenarios. ( d ) Probe transmission as function of probe detuning for the three different pump scenarios described in c , through the plasmonic–atomic device. ( e ) Probe transmission through the reference cell. In both panels ( d , e ), the green line represents the case where the pump beam is tuned far from resonance, the blue line represents the pump beam tuned to the F =2 to F ′ manifold, and the red lines represent tuning the pump to F =3 to F ′ manifold. Full size image Next, we describe the level scheme and general transmission in such systems in the framework of velocity-selective optical pumping. In Fig. 6b , we describe the 85 Rb D1 and D2 hyperfine manifolds. The pump beam, when is tuned to resonance from the F =3 ground state to the F ′ manifold, is in resonance with three different velocity groups, depending in its specific detuning from each F ′=2,3,4 hyperfine levels. Thus, the probe beam is expected to experience reduced absorption at these specific velocity groups. As the probes beam manifold consists of two hyperfine levels, we expect to see overall six Doppler-free line shapes. As a result, one can measure the hyperfine manifold of both the D1 and D2 lines simultaneously. Another prominent advantage of this technique is the ability to achieve Doppler-free lines with copropagating beams, assisting the ability to couple easily into apparatuses utilizing atoms and guided propagating modes. Subsequently, we turn to describe the experimental results. First, we tune to the prism to an angle around the plasmonic resonance. Next, we scan the probe across the F =3 to F ′ manifold while the pump is far from resonance, and thus does not influence the atomic system whatsoever. This is illustrated in Fig. 6c (middle panel) in green. The obtained lineshape is shown in Fig. 6d,e (green lines), for both the plasmonic–atomic device ( Fig. 6d ) and the reference cell ( Fig. 6e ). One can easily notice a peak in transmission, corresponding to the Fano response discussed earlier in the text. Next, we tune the pump to resonance with the D2 F =3 to F ′ manifold (illustrated in left panel of Fig. 6c , in red). As the atoms are now pumped out of the F =3 level, we expect and indeed obtain an increase in transmission of the probe beam through the reference system at specific frequencies corresponding to three selected velocity groups ( Fig. 6e , red line). However, for our plasmonic–atomic system, we instead obtain a decrease in the probes transmission. ( Fig. 6d , red line). This is a direct result of the Fano effect which inverts the transmission characteristics around resonance. The important capability to almost switch off the Fano lineshape and obtain a flat transmission spectrum is believed to be a result of the high energy density in the plasmonic mode. Quantitatively, this result was obtained with estimated pump intensities of 15 W cm −2 in the plasmonic system (compare with unsaturated power levels for the reference system). The large intensity value is a direct result of the well known [20] , [40] , [41] , local field energy enhancement (the MgF 2 , being only 5-nm thick, has a negligible effect on the enhancement), which is typical for plasmonic systems. For the specific conditions of our experiment, twofold increase in the intensity is calculated. One should note, that in comparison with a bare glass-attenuated total internal reflection apparatus, the intensity enhancement is of the order of ~20, consistent with previously reported near field measurements [41] . We believe that as a consequence of this intensity enhancement, the transitions obtained in our hybrid plasmonic–atomic system are highly saturated and power broadened, resulting in a reduction in contrast over a broad spectral regime. Finally, when we tune to pump to resonance with the F =2 to F ′ manifold (illustrated in right panel of Fig. 6c , in blue), we obtain the opposite scenario. As additional atoms are now pumped into of the F =3 level via transition from the excited states, we expect and indeed obtain a decrease in transmission of the probe beam through the reference system at specific frequencies corresponding to three selected velocity groups ( Fig. 6e , blue line). Again, for our plasmonic–atomic system, the effect is inverted and instead we obtain an increase in the probe transmission ( Fig. 6d , blue line). As a final comment, we note that we were also able to witness Doppler-free signals not only in the reference cell but also in our atomic–plasmonic devices, with line widths of few tens of MHz. This work is still in progress and a detailed report on these observations will be given elsewhere. We have developed a hybrid atomic–plasmonic resonant system and observed light–matter interactions between SPP modes and absorption lines of an atomic vapour. The coupling between plasmonic and atomic resonances produces spectroscopic line shapes that cannot be obtained by each of the individual components and materials. Here, simply by changing the phase-matching conditions, we control the interplay between plasmonic and atomic resonances at will. This degree of freedom allows the achievement of both symmetric and antisymmetric line shapes, and to observe the gradual evolution of these states. Furthermore, the coupling between atomic and plasmonic resonances gives rise to a Fano-type response. In addition to the fundamental aspects related to the phenomena of Fano resonance, the interaction of a plasmonic system with atomic vapour such as Rb is very appealing due to the myriad applications that have been demonstrated using alkali vapours in the past decades [42] , [43] , [44] , [45] . Indeed, the community has vast experience in manipulating and controlling such vapours close to room temperature, using both linear and nonlinear interrogation techniques. In the quest for miniaturization, plasmonic and atomic vapour interactions hold a great promise to shed light on the basic nature of light–matter interactions between surfaces and atoms due to the unprecedented light concentration in plasmonic structures [23] . As a consequence, it is possible to design plasmonic structures that interact with atoms in the very close vicinity of the vapour–metal surface [21] , where surface interactions of few tens of nanometers [38] , [39] may be measured in plasmonic systems. Additionally, given that plasmonic systems can be tailored to operate over a wide spectral band, our platform can also be applied to other transitions in Rb as well as in other alkali vapours such as caesium, potassium and sodium. For example, easier probing of surface effects is expected by operating at higher optical frequencies, in the vicinity of the blue portion of the spectrum (for example, at the 5 2 S 1/2 to 6 2 P 3/2 secondary transition at 420 nm). Such operation is anticipated to be of high importance in the investigation of Rydberg [42] states, in the vicinity of metals. Furthermore, understanding the nature of light–matter interactions along metal surfaces may assist the realization of cold atoms chips [21] , [38] , [46] in which better understanding of surface interactions is crucial. The research of the basic behaviour of atoms near different surfaces, holds great promise for developing miniaturized plasmonic–atomic vapour-based devices for applications such all-optical switching [43] benefiting from the strong field confinement in such systems. The enhanced sensitivity provided by the plasmonic resonance can also be used for metrology applications, for example, magnetometers [44] , frequency standards [45] and encoders. For instance, it has been recently demonstrated that using evanescent wavelengths and 100-μm coated cells, one can measure magnetic fields in the pT level [47] . Additional potential applications are few photon switching [48] , pulse shaping [49] and myriad of other nonlinear optical effects. As an example for a potential application, we have demonstrated the ability to obtain efficient all-optical control of light transmission with relatively low powers. Improvements in contrast and in switching power can be achieved, for example, using higher density of atoms and localized plasmons such as nanoantennas [21] . Finally, a prime interest of our future research will be devoted for observing strong coupling effects in our system. While our simulations predict some degree of resonance splitting, it was extremely difficult to observe this effect in our current experiment. Future experimental work will be devoted to investigate the resonance splitting as a function of temperature. Furthermore, by replacing the thin metallic film with other plasmonic structures, we may achieve higher localized density of states with the end result of stronger resonance splitting. Device fabrication To construct the device, we use a BK7 right-angle prism (Foctek Photonics), which is coated by a 3-nm adhesion layer of Ti, a 42-nm layer of Au and a 5-nm-thick passivation layer of MgF 2 using thermal evaporation. The role of the upper MgF 2 layer is to protect the gold layer from interacting with the Rb atoms. Finally, a Pyrex cylinder is bonded to the chip using thermally cured epoxy. The cell is connected to a turbo vacuum system, and baked out simultaneously. The device is baked out for 24 h after which a vacuum level of at least 10 −7 Torr is reached. At this stage, 85 Rb is inserted into the cell, and the cell is disconnected and sealed. Optical setup A 780-nm DFB (Newport 2010M) laser source illuminates the fabricated device which is mounted on a rotation stage. The transmission is measured using a photodetector (Thorlabs DET100A). The intensity of the launched light is controlled by neutral density filters positioned at the output of the laser. In addition, a beam splitter is placed in the output of the laser for the purpose of measuring a reference cell (with natural Rb). In the all-optical control experiment, we use an additional laser (D1 line 795 nm, Toptica DL100). To separate between the copropagating 780 and 795 nm beams, we use a blazed, ruled grating (TL GR13-1208). To achieve sufficient density of atoms, the device is heated using resistor heaters, and the temperature is monitored using a thermistor, which is located a few millimeters from the top of the cell. To reduce the accumulation of Rb on the gold surface, we maintain a temperature gradient between the top of the cylinder and the surface. This way, the Rb droplet is created at the top of the cylinder, where the temperature is lower. How to cite this article: Stern, L. et al. Fano resonances and all-optical switching in a resonantly coupled plasmonic–atomic system. Nat. Commun. 5:4865 doi: 10.1038/ncomms5865 (2014).